Taking snapshots of photosynthetic water oxidation using femtosecond X-ray diffraction and spectroscopy The dioxygen we breathe is formed by light-induced oxidation of water in photosystem II. O 2 formation takes place at a catalytic manganese cluster within milliseconds after the photosystem II reaction centre is excited by three single-turnover flashes. Here we present combined X-ray emission spectra and diffraction data of 2-flash (2F) and 3-flash (3F) photosystem II samples, and of a transient 3F’ state (250 μs after the third flash), collected under functional conditions using an X-ray free electron laser. The spectra show that the initial O–O bond formation, coupled to Mn reduction, does not yet occur within 250 μs after the third flash. Diffraction data of all states studied exhibit an anomalous scattering signal from Mn but show no significant structural changes at the present resolution of 4.5 Å. This study represents the initial frames in a molecular movie of the structural changes during the catalytic reaction in photosystem II. Aerobic life on earth is supported by the constant regeneration of dioxygen through photosynthetic water oxidation in green plants, algae and cyanobacteria. This reaction takes place in photosystem II (PS II), a multi-subunit membrane protein complex. PS II couples the one-electron photochemistry of the primary charge separation at the reaction center with the four-electron redox chemistry of water oxidation at the Mn 4 O 5 Ca cluster of the oxygen evolving complex (OEC) at the lumenal side of the protein complex, using the spatial and temporal organization of the electron donor and acceptor cofactors in PS II [1] , [2] . This well-controlled electron and proton flow results in the high quantum efficiency of PS II. During the water oxidation reaction, the OEC functions as a redox capacitor by storing four oxidizing equivalents before the release of molecular oxygen. Starting from the dark stable S 1 state, the oxidation state of the OEC is increased by one on each light excitation of PS II until the highest oxidized stable intermediate state, S 3 , is reached. Following the next light excitation, the OEC is oxidized one more time to form the transient S 3 Y Z ox and S 4 states that lead to dioxygen formation, which converts the OEC to its most reduced state, S 0 (ref. 3 ). The fourth light excitation sets the OEC back to the S 1 state, and thereby completes the cycle ( Fig. 1a ). 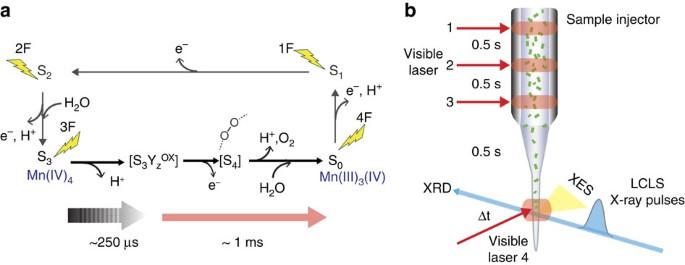Figure 1: Flash-induced changes in PS II and experimental set-up used at LCLS. (a) Kok cycle describing the different stable intermediate states of the catalytic water oxidation reaction in PS II. (b) Scheme for the illumination set-up used to advance PS II in the catalytic cycle and measure simultaneously the XRD and XES signal at LCLS. Lasers 2 and 3 were used to generate 2F samples, lasers 1, 2 and 3 for 3F samples and lasers 2, 3 and 4 to generate the 3F’ samples. Figure 1: Flash-induced changes in PS II and experimental set-up used at LCLS. ( a ) Kok cycle describing the different stable intermediate states of the catalytic water oxidation reaction in PS II. ( b ) Scheme for the illumination set-up used to advance PS II in the catalytic cycle and measure simultaneously the XRD and XES signal at LCLS. Lasers 2 and 3 were used to generate 2F samples, lasers 1, 2 and 3 for 3F samples and lasers 2, 3 and 4 to generate the 3F’ samples. Full size image Much structural and mechanistic information about PS II, the OEC and the O–O bond formation was gained through mass spectrometric [4] , various spectroscopic [4] , [5] , [6] , [7] , [8] , [9] , crystallographic [10] , [11] , [12] , [13] and theoretical [14] , [15] , [16] studies over the past decade. In particular, the most recent structure, inferred from X-ray diffraction (XRD) data, has provided detailed geometric information of the OEC, including ligands and bound water molecules [13] . Most of the experimental studies, however, are carried out at cryogenic temperatures and represent a static picture of the system in a frozen state. Although the stable intermediate states, S 0 through S 3 , can be trapped and studied at cryogenic temperatures, the critical S 3 → S 3 Y Z ox → S 4 → S 0 step—where dioxygen is formed, two protons and O 2 are released, and where at least one substrate water binds—only occurs under ambient conditions and has no intermediates that can be cryotrapped. To date, there has been only one transient X-ray spectroscopy study of the S 3 → S 3 Y Z ox → S 4 → S 0 transition performed at room temperature (RT) [17] . More detailed investigations of the transient states by X-ray spectroscopy and by kinetic crystallography have been hampered due to the severe radiation damage, especially to the Mn 4 CaO 5 cluster that is significantly faster at RT as compared with cryogenic conditions. However, X-ray-induced changes, particularly at the redox-active metal site, have even been an issue for experiments carried out at cryogenic temperatures [18] , [19] , [20] . We have recently introduced a combined spectroscopy and diffraction data collection methodology at RT [21] using the ‘probe before destroy’ method [22] , [23] , [24] made possible by the ultra-short (fs) and bright X-ray pulses of an X-ray free electron laser (XFEL). In this approach, XRD data and Mn Kβ-X-ray emission spectra (XES), sensitive to the metal charge density [25] , [26] , are measured simultaneously from micrometre-sized crystals of PS II, thereby obtaining information about the geometric and the electronic structure of the active site, under identical conditions. Owing to the ultra-short fs X-ray pulse duration, the sample is probed before the manifestation of X-ray induced changes—which predominantly take place on the picosecond time scale (for damage to the atomic structure)—even under ambient conditions. One should note that with conventional synchrotron X-ray sources the main source of radiation damage is via the generation of radicals from the solvent (water). Subsequent diffusion of these radicals leads to specific damage (for example, reduction of metal sites) and modification of amino acid side chains (for example, decarboxylations). Such events are diffusion controlled and occur on a longer time scale (>picoseconds) and seem not to be dependent on the dose rate. Earlier work [21] , [27] showed that the approach of using ultrafast (<50 fs) and ultra-bright (10 12 photons per pulse) X-ray pulses permits the collection of XES and XRD data from intact PS II, and we reported results from the dark-adapted ( S 1 ) and the one flash ( S 2 ) samples with an XRD resolution limited to 5.5 Å. Here we present XES and XRD data from the last step of the Kok cycle, where O 2 is evolved, with an improved resolution of 4.5 Å. This step, triggered by the third flash given to dark-adapted PS II samples, advances the PS II complex from the S 3 to the S 0 state, via the transient S 3 Y Z ox and S 4 states ( S 3 → S 3 Y Z ox → S 4 → S 0 transition). Furthermore, we observe an anomalous signal for the Mn atoms in the OEC from all the states, including the transient S 3 Y Z ox state. This observation supports the quality of our XRD data and also the data analysis protocols, and we envision that the Mn anomalous signal could be used as a sensitive probe for monitoring changes of the atomic positions of Mn in the OEC during the catalytic cycle in future studies at higher resolution. XES at different time points in the catalytic cycle PS II was advanced through its reaction cycle in situ , using a flow/illumination scheme ( Fig. 1b ) employing an electrospun liquid jet [28] . The protocol consisted of visible-laser illumination using three optical fibres directly attached to the sample delivery capillary, and an additional laser for illumination of the sample in the jet (see Methods). The temporal frequency for illumination was chosen to match the sample flow rate, so that each volume segment was illuminated by each fibre once while passing through the capillary. The set-up also allows enough time (~0.5 s) for complete PS II turnover between consecutive illuminations, which takes into account the slower acceptor side reactions [7] , [29] , [30] , [31] , while being rapid enough to avoid significant decay of the S -states, that are stable for on the order of several tenth of seconds. The fourth laser (labelled ‘laser 4’ in Fig. 1b ) illuminated the sample in the jet, to study transients during the S 3 to S 0 transition by changing the timing between the third visible-laser pulse and the X-ray probe pulse. O 2 detection via membrane-inlet mass spectrometry (MIMS) was used for optimizing the conditions for S -state turnover in the capillary flow sample delivery system, using a facsimile of the flow/illumination set-up employed at Linac Coherent Light Source (LCLS) (see Methods). One of the most important factors in the illumination scheme is the required light intensity for efficient turnover through the S i state cycle. Too low intensities can lead to only partial turnover of the samples, while too high intensities increase the miss parameter via light scattering along the capillary, and may also inactivate the sample. The optimal light intensity can be found by the quality of the O 2 oscillation pattern, and also by the total O 2 produced per PSII complex and flash number. The former method should normally be sufficient, but a small uncertainty remains whether there can be a certain part of the sample that never sees any light, and thus does not contribute to the oscillation pattern. To address this question, the latter method needs to be employed (see Methods), which requires the absolute calibration of the MIMS signals. The amount of 0.73 O 2 /RC after three flashes ( Fig. 2a ) shows that the light conditions used for illumination are optimal for saturating all PSII reaction centres in the sample. The O 2 evolution patterns obtained from PS II solutions and PS II microcrystals ( Fig. 2b ) show light-induced turnover of the catalytic cycle as expected. Analysis of the flash pattern indicates that the S 3 state is the majority component (≥55%) in the samples given two visible-laser flashes (2F) with virtually no S 0 state present. In contrast, the largest component in the 3F samples is the S 0 state (≥40%). Therefore, the difference between the 3F and 2F samples is dominated by the formation of the S 0 state at the expense of the S 3 state. 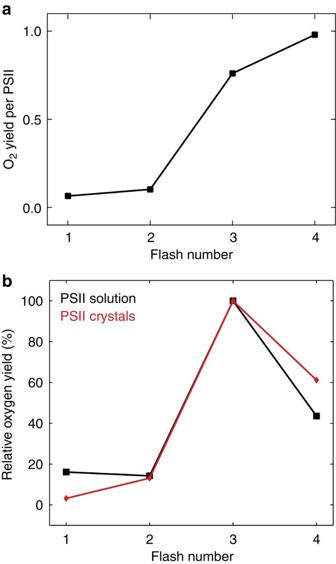Figure 2: Oxygen production by PSII. (a) O2yield per PSII reaction centre as detected by MIMS as a function of flash number (measurement shown is for PS II solutions, flow rate 0.5 μl min−1, frequency 4 Hz, light intensity was 7 μJ for each fibre). (b) O2yield measured by MIMS as a function of flash number from PS II solutions (black) and PS II microcrystals (red). Figure 2: Oxygen production by PSII. ( a ) O 2 yield per PSII reaction centre as detected by MIMS as a function of flash number (measurement shown is for PS II solutions, flow rate 0.5 μl min −1 , frequency 4 Hz, light intensity was 7 μJ for each fibre). ( b ) O 2 yield measured by MIMS as a function of flash number from PS II solutions (black) and PS II microcrystals (red). Full size image We measured XES on PS II solutions at the Coherent X-ray Imaging (CXI) instrument [32] at LCLS (see Methods). As shown in Fig. 3 , a clear shift between the 2F ( S 3 -enriched) and 3F ( S 0 -enriched) spectra is observable. Calculation of the first moment (see Methods) revealed that the 3F spectrum is shifted ~0.1 eV to higher energies indicating a reduction of Mn [26] , as expected for the transition of the OEC from the highly oxidized S 3 to the most reduced S 0 state, in which the formal oxidation states are assigned as Mn 4 IV and Mn 3 III Mn IV , respectively [1] , [2] , [6] , [33] , [34] . Comparing these data to synchrotron radiation (SR) data collected at cryogenic temperature from Thermosynechococcus elongatus PS II and previously recorded data from spinach PS II [35] shows a very similar trend ( Fig. 3c and Supplementary Fig. 1 ). 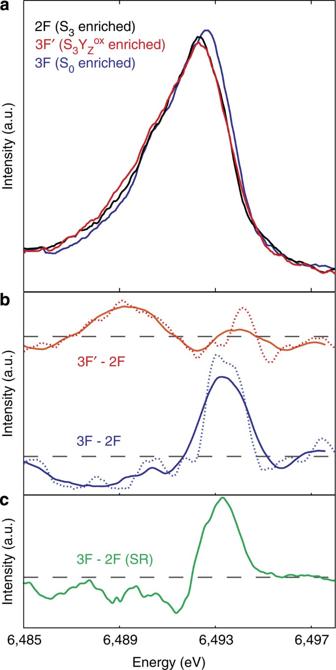Figure 3: Mn Kβ XES of PS II. (a) XES recorded with <50 fs X-ray pulses at LCLS. Spectra were measured 0.5 s after two laser flashes (2F, black; lasers 2 and 3 on), or 0.5 s after three laser flashes (3F, blue; lasers 1, 2 and 3 on), and ~250 μs after three laser flashes (3F’, red; lasers 2, 3 and 4 on), respectively. (b) Difference between the Mn Kβ XES of PS II, blue: 3F–2F; red: 3F’–2F. Before calculating the difference curves, spectra were smoothed by moving average (dotted line) or cubic polynomial fitting (solid line, similar to the procedure used for analysing the synchrotron data). (c) The 3F–2F difference spectrum (green) from SR data collected at 15 K. Figure 3: Mn Kβ XES of PS II. ( a ) XES recorded with <50 fs X-ray pulses at LCLS. Spectra were measured 0.5 s after two laser flashes (2F, black; lasers 2 and 3 on), or 0.5 s after three laser flashes (3F, blue; lasers 1, 2 and 3 on), and ~250 μs after three laser flashes (3F’, red; lasers 2, 3 and 4 on), respectively. ( b ) Difference between the Mn Kβ XES of PS II, blue: 3F–2F; red: 3F’–2F. Before calculating the difference curves, spectra were smoothed by moving average (dotted line) or cubic polynomial fitting (solid line, similar to the procedure used for analysing the synchrotron data). ( c ) The 3F–2F difference spectrum (green) from SR data collected at 15 K. Full size image In addition to the 2F and 3F spectra, we measured the XES at a time point 250 μs after the third flash (3F′) using lasers 2, 3 and 4 ( Fig. 1 ). The XES for this transient state is similar in position to the 2F spectrum ( Fig. 3a,b ), but its shape is different with broadening towards the lower energy side. Although such broadening could be caused by oxidation of a fraction of the lower S -states ( S 1 and S 2 ) in our sample, it could also be due to light-induced changes in the electronic structure of the S 3 fraction. Nevertheless, the result shows that there is no significant reduction or oxidation of the Mn taking place within the 250-μs time span between the third visible-laser excitation pulse and the X-ray probe pulse. XRD in the higher S -states XRD data from 2F ( S 3 -enriched), 3F ( S 0 -enriched) and 3F′ ( S 3 Y Z ox -enriched; 250 μs after the third flash) PS II crystals, as well as in the dark state ( S 1 ), were collected. Microcrystals of PS II were prepared using a new seeding protocol (see Methods). Clear Bragg spots were observed to a resolution of ~4.1 Å, with thermal diffuse scattering extending well beyond this to ~3.0 Å, indicative of correlated atomic motion in the crystal. For the 2F data, a total of 16,973 indexed patterns were merged resulting in a data set of 4.5 Å resolution (see Table 1 and Supplementary Tables 1 and 2 for details). The resolution cutoff for the merged data sets was chosen based on the resolution dependence both of the multiplicity and of CC 1/2 , the correlation coefficient of semi-data sets merged from odd- and even-numbered images [36] ; that is, completeness >90%, multiplicity >6 and CC 1/2 >30%. Likewise, data sets of 3F, 3F’ and 0F states were obtained with resolutions of 4.6 Å (13,094 lattices), 5.2 Å (7,850 lattices) and 4.9 Å (6,695 lattices), respectively ( Table 1 and Supplementary Tables 1 and 3–5 ). Electron density maps for all four states are shown in Fig. 4 and Supplementary Figs 2 and 3 . A comparison with the SR data cut to the same resolution shows that the level of detail visible is as expected for this resolution range ( Supplementary Fig. 4 ). The occupancy for selected non-protein molecules was set to zero and the simulated annealing omit maps were computed for all data sets, to remove potential model bias arising from phasing with a complete, high-resolution starting model (pdb: 3bz1) [12] . The result clearly shows the electron density of the Mn 4 O 5 Ca cluster, the non-haem Fe, the chlorophyll and even partially for the quinone cofactors ( Supplementary Fig. 3 ) in the mF o −DF c difference maps. The regions around the OEC, the acceptor-side quinones and non-haem iron, where the largest changes are expected, were inspected for changes between the different states. No statistically significant changes were observed in the 2 mF o −DF c maps of the individual data sets ( Fig. 4a,b and Supplementary Figs 2 and 3 ) and in the isomorphous difference maps ( mF o −mF o ) between the different data sets ( Fig. 4c,d and Supplementary Fig. 5 ). This shows that any structural changes related to the S -state transitions are smaller than what we can detect at the current resolution. However, it should be noted that the mF o −DF c Fourier maps contain several features that are observed consistently in both monomers and all flash states; namely, an electron density peak at the position of the OEC when viewed at a contour level of +3 σ , a small peak 10 Å distant that appears to be coordinated by residues Glu 333 and Asp 61 of the D1 polypeptide, and other nearby peaks. Smaller negative peaks are seen at the −3 σ contour, for example, close to Val 185 and Phe 182 of the D1 protein ( Supplementary Fig. 6 ). In general, we observe these low-intensity peaks at the same positions in both monomers and across all four illuminated states. This suggests that they are not artefacts of the Fourier transform, and are rather due to structural differences between SR data collected at cryogenic temperature and the RT data presented here. However, the current resolution does not allow them to be fully modelled in our final atomic coordinate sets. Table 1 Statistics for processed data and refined structures. 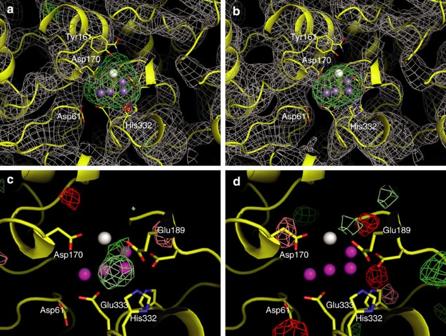Figure 4: Electron density maps obtained for PS II. (a) 2mFo−DFcmaps for the dark and (b) the 2F data of PS II are shown in grey contoured at 1.0σ,mFo−DFcmaps after omitting the OEC are shown in green and red, contoured at ±5.0σ. (c)mFo−mFoisomorphous difference maps for the 2F–dark data and (d) the 3F–2F data are shown for both monomers and are contoured at +3σ(bright green, monomer I; pale green, monomer II) and −3σ(red, monomer I; salmon, monomer II) together with the model for the 2F data (Mn shown as magenta spheres, Ca as white sphere). Full size table Figure 4: Electron density maps obtained for PS II. ( a ) 2 mF o −DF c maps for the dark and ( b ) the 2F data of PS II are shown in grey contoured at 1.0 σ , mF o −DF c maps after omitting the OEC are shown in green and red, contoured at ±5.0 σ . ( c ) mF o −mF o isomorphous difference maps for the 2F–dark data and ( d ) the 3F–2F data are shown for both monomers and are contoured at +3 σ (bright green, monomer I; pale green, monomer II) and −3 σ (red, monomer I; salmon, monomer II) together with the model for the 2F data (Mn shown as magenta spheres, Ca as white sphere). Full size image Measurement of anomalous XRD signal from Mn in PS II Accurate determination of the Bragg spot intensities and the derived structure factors is challenging for single-shot crystallography at XFELs [21] , [23] , [24] . As a control to validate the data quality and our analysis protocol, we investigated whether small anomalous differences could be detected in the recorded Bragg spot intensities. Such differences between inversion-related Bragg spots (Bijvoet pairs) arise from the collection of diffraction data at energies above an absorption edge and are often only in the order of ~1% of the total signal intensity. We used an incident energy of 7.1 keV in our current XES/XRD data collection, which is close to the Mn edge (6.54 keV), and favours observing the anomalous signal from Mn in the OEC. As a positive control of the methodology, we first analysed microcrystal diffraction data from a model system, thermolysin, which natively binds one Zn and several Ca ions [37] . Data from thermolysin microcrystals were collected at 1.27 Å (9.76 keV), ~100 eV above the Zn edge (9.66 keV). Diffraction was observed out to the corners of the detector (1.50 Å) and the integrated intensities were merged to obtain a data set to 1.80 Å resolution ( Table 1 and Supplementary Table 6 ). 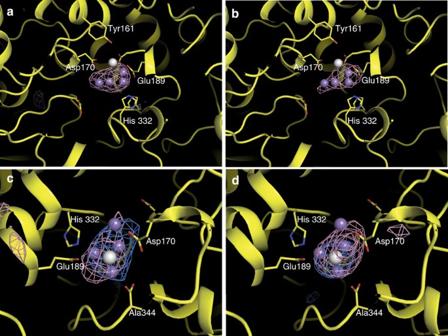Figure 6:Anomalous signal from Mn for different illumination states of PS II. (a) Anomalous map of the OEC in PS II is shown for the 2F data (magenta) in monomer I. (b) Anomalous map of the 3F data in monomer I. (c) Anomalous map of the 2F (cyan) and 3F (magenta) data in monomer I, orientation is rotated by 90° around horizontal and vertical axis compared with the view ina. (d) Anomalous map for monomer II, 2F (cyan) and 3F (magenta) data are shown, view direction is similar toc. All maps shown are anomalous difference simulated annealing omit maps contoured at 3σ. Analysis of the Bijvoet pairs in the merged data showed a clear anomalous signal contribution, and anomalous difference maps showed a clear maximum, 18 σ above the mean, located at the position of the Zn ion as well as lower maxima for three of the four Ca ions and for the sulphur of one of the methionine residues ( Fig. 5a,b and Supplementary Fig. 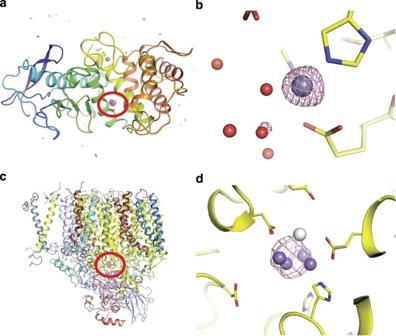7 ). Figure 5: Anomalous signal in the XFEL data sets. (a) Anomalous difference map of the thermolysin data after simulated annealing with the occupancy for Zn and Ca set to zero to minimize model bias. The map is contoured at 4.0σ, extending over the entire thermolysin molecule. The position of the highest peak in the map (Zn atom) is highlighted. (b) The same anomalous difference map of thermolysin shown in the region of the natively bound Zn ion (magenta sphere), contour level at 3.0σ. (c) Anomalous difference map obtained from the 3F data of PS II, shown for one monomer, location of the strongest peak is highlighted, contour level at 4.0σ. (d) Enlarged view of the 3F anomalous density for the region of the OEC (contoured at 4.0σ; Mn shown as magenta spheres, Ca as white sphere). All maps shown are anomalous difference simulated annealing omit maps. Figure 5: Anomalous signal in the XFEL data sets. ( a ) Anomalous difference map of the thermolysin data after simulated annealing with the occupancy for Zn and Ca set to zero to minimize model bias. The map is contoured at 4.0 σ , extending over the entire thermolysin molecule. The position of the highest peak in the map (Zn atom) is highlighted. ( b ) The same anomalous difference map of thermolysin shown in the region of the natively bound Zn ion (magenta sphere), contour level at 3.0 σ . ( c ) Anomalous difference map obtained from the 3F data of PS II, shown for one monomer, location of the strongest peak is highlighted, contour level at 4.0 σ . ( d ) Enlarged view of the 3F anomalous density for the region of the OEC (contoured at 4.0 σ ; Mn shown as magenta spheres, Ca as white sphere). All maps shown are anomalous difference simulated annealing omit maps. Full size image In PS II, a clear anomalous signal ( Fig. 5c,d , Fig. 6 and Supplementary Figs 8 and 9 ) from Mn in the OEC is also detected in all four data sets (0F, 2F, 3F and 3F′) ( Supplementary Table S1 ). Figure 5c,d shows the anomalous difference map from the 3F data after omitting the OEC and performing simulated annealing refinement. It is evident from the overview shown in Fig. 5c that the largest peak ( σ >6) in the anomalous density is located at the position of the OEC. The density covers the Mn ions in the cluster and does not include the Ca ( Fig. 5d ) as expected from the weaker anomalous contribution of Ca at 7.1 keV ( f ″ of 1.6 for Ca compared with 3.4 for Mn at 7.1 keV). Similar results were obtained for the other PS II data sets for both monomers in the PS II dimer ( Fig. 6 and Supplementary Figs 8 and 9 ). It should be noted however that the anomalous difference Patterson maps did not reveal peaks above the noise level attributable to Mn. This result is expected as also the anomalous data measured at SR sources at 3.5 Å resolution [10] did not yield any peaks in the Patterson map above the noise level, due to the large protein mass and the low number of anomalous scatterers per unit cell volume. Figure 6: Anomalous signal from Mn for different illumination states of PS II . ( a ) Anomalous map of the OEC in PS II is shown for the 2F data (magenta) in monomer I. ( b ) Anomalous map of the 3F data in monomer I. ( c ) Anomalous map of the 2F (cyan) and 3F (magenta) data in monomer I, orientation is rotated by 90° around horizontal and vertical axis compared with the view in a . ( d ) Anomalous map for monomer II, 2F (cyan) and 3F (magenta) data are shown, view direction is similar to c . All maps shown are anomalous difference simulated annealing omit maps contoured at 3 σ . Full size image The quality of the PS II XRD data reported here for the S 1 state is improved compared with the previously obtained XFEL data: 4.5 Å versus 5.7 Å [21] . Owing to the inherent fluctuations in pulse intensity, crystal size and crystal quality in single-shot microcrystal experiments at an XFEL, the signal strength varies from shot to shot. Therefore, we expect a distribution of diffraction images with different maximum resolution. To avoid adding noise into the diffraction data, an individual resolution cutoff was computed for each diffraction image based on the signal strength (see Methods). The observed distribution of the resolution for PS II as well as for thermolysin explains why the multiplicity in both cases ( Supplementary Tables 2–6 ) decreases steadily in the higher resolution shells. Recently, the first observation of an anomalous signal from femtosecond diffraction experiments with microcrystals at an XFEL [38] and the first successful de novo phasing of lysozyme at 2.1 Å resolution using the anomalous signal of gadolinium obtained in an XFEL experiment were reported [39] . In the gadolinium phasing experiment of lysozyme, the anomalous signal strength was around 5–15% [39] . In comparison, we expect an anomalous signal of <1% for Mn in PS II and of ~1.5% for Zn in thermolysin. The observation of the very strong anomalous peak for Zn in the thermolysin data indicates that the Bragg peak intensities were determined with sufficient accuracy to extract the weak anomalous difference (see ref. 40 for a report on determining the anomalous Zn signal of thermolysin from SR measurements). Furthermore, the presence of the anomalous density for Mn in all of the PS II data sets, despite the expected low signal strength, confirms the quality of the data and implies that structure factors can be extracted reliably from the current PS II data sets. In this regard, it should be noted that even the high-resolution shell of the data still contains a considerable amount of anomalous signal as can be seen in Supplementary Fig. 9B . As described above, the electron density of PS II shows the level of detail expected at the specified resolutions (4.5–5.2 Å, depending on number of collected images per S -state; Supplementary Fig. 4 ). The quinone co-factors ( Q A in the dark, 2F and 3F data; Q B in the 3F data), that were not visible in the previous XFEL data due to limited resolution, are now partially visible in the mF o −DF c difference maps ( Supplementary Fig. 3 ). In the earlier SR XRD structures of PS II [10] , [41] , [42] , [43] , [44] with a resolution lower than 3.0 Å, it was difficult to locate them with confidence (especially the mobile Q B ) due to partial occupancy and quinone mobility. The native XRD data indicate that there are no large-scale rearrangements of the Mn 4 O 5 Ca cluster and its protein environment between the different states (dark, 2F, 3F and 3F′) in PS II. This is in line with Mn EXAFS data, which suggests that the largest possible changes in Mn–Mn distances on S -state transitions are <0.5 Å (this estimate is based on the changes proposed in the S 2 to S 3 transition, if di-μ-oxo bridged Mn becomes mono-μ-oxo bridged) [20] , which are well below the sensitivity of our current XRD measurements. To test the level of change detectable using our data, we simulated a shift of the Mn 4 CaO 5 cluster by 1 and 0.4 Å compared with the starting model based on SR data. In both cases, a strong positive and negative peak corresponding to the shift was visible in the isomorphous difference density ( Supplementary Fig. 10A,B ), indicating that shifts of that magnitude should be detectable within the signal to noise level of the current data. In contrast, when only perturbing the position of a single Mn within the Mn 4 CaO 5 cluster by 0.5 Å, no clear peaks were observed in the difference density ( Supplementary Fig. 10C ), indicating that a structural change of such order can not be resolved at the present resolution. We furthermore evaluated the noise level in the current electron densities by computing the difference in position of the Mn 4 CaO 5 cluster between the two monomers in each data set. For this approach, we superimposed the mF o −DF c Fourier omit maps after simulated annealing (see Methods) for the two monomers and evaluated the differences between the OEC peak in these maps. The values are in the range of 0.3–0.6 Å, indicating that changes in Mn positions larger than ~0.5 Å should be visible in our data. The height and volume of the anomalous XRD difference map peak of the OEC reflects the amount of data available for each S -state data set. Supplementary Fig. 9A shows that after scaling the anomalous difference densities of the 2F, 3F and 3F′ data sets individually at a σ -value of 80% of the peak maxima, the extent of the anomalous peak at the OEC is roughly similar for all data sets. It is also evident from this plot that the peak position of the anomalous signal for all data sets is in the vicinity of the centre of mass of the four manganese, as expected for a signal originating from Mn. Before attempting to interpret the visible differences in the anomalous signal for the different S -states in terms of structural differences of the Mn 4 CaO 5 cluster, it should be noted that at the present resolution the difference of the anomalous signal between two monomers in one PS II dimer is larger than the differences for the Mn 4 CaO 5 cluster in the same monomer in different S -states. We quantified this by evaluating the difference in the peak position for the OEC between the two monomers for each of the data sets and found differences in the order of above 1 Å. This indicates that the noise level in our present anomalous data precludes the observation of the small changes expected between the different illumination states. Therefore, analysis of detailed structural changes based on the anomalous signal of the OEC has to await higher data quality, and in the light of the present data interpretations of structural changes can only be made using the isomorphous omit maps, as these are derived from the full data for each flash state instead of only the anomalous data and consequently show lower noise levels. We have used fs XES to follow the changes in the oxidation state of the Mn 4 CaO 5 cluster on advancing from the S 3 to the S 0 state. The peak shift that was observed between the 2F and the 3F sample reproduced the shift in oxidation state between the highest oxidized ( S 3 state) and most reduced state ( S 0 state) found earlier [35] . Interestingly, the peak position of the spectrum observed at the transient time point, 250 μs after the third flash, is very similar to that of the 2F spectrum. The observation that there is no significant change in the oxidation state of Mn within this time span is consistent with the kinetics of Mn oxidation/reduction in the S 3 → S 3 Y Z ox → S 4 → S 0 transition based on earlier time-resolved ultraviolet–visible [45] , [46] , electron paramagnetic resonance [47] , infrared spectroscopy [7] and Mn K-edge XAS [17] studies. It was inferred from these studies that a de-protonation step, forming a transient state S 3 Y Z Ox ,(also refered to as S 3 ′) [7] , [46] occurs before Mn redox chemistry [7] , [46] . This lag phase before the onset of Mn redox chemistry was reported to be in the range of 100–250 μs [7] , [17] . Our results provide direct evidence that Mn redox chemistry does not occur within the first 250 μs after illumination of the S 3 state. This implies that the formation of a Mn V species that has been invoked for a nucleophilic attack mechanism [2] , or the formation of a peroxide intermediate that will result in Mn reduction [1] , does not occur within the first 250 μs after the third flash. The formation of an oxygen radical species [4] , [6] within this time period cannot be excluded by our data (as no Mn oxidation would be involved), but is unlikely on the basis of the earlier ultraviolet–visible data [45] . The long delay before the onset of Mn redox chemistry suggests that the formation of the S 3 Y Z ox state is not a simple deprotonation step. It is rather likely to be accompanied by slower structural changes of the Mn 4 CaO 5 cluster and/or the protein framework [7] that are required to stabilize the deprotonated S 3 Y Z ox state of the OEC in the conformation necessary for subsequent O–O bond formation. In line with this conclusion, a recent report [46] underlined the importance of the exact structure of the H-bonding network for efficient turn over in the S 3 → S 3 Y Z ox → S 4 → S 0 transition by demonstrating that Ca/Sr exchange in the OEC perturbs the H-bonding network and results in a significant slowing of the S 3 → S 3 Y Z ox transition [4] , [46] . In summary, we have investigated the S -state intermediates and a transient state with fs XES/XRD by following the S -state transitions under ambient conditions. Advancement of S -states by in situ photoexcitation was confirmed by the O 2 evolution pattern and the XES spectral shifts. The XES data indicate that the Mn oxidation state does not change within 250 μs after the illumination of the S 3 state. The most probable explanation for this observation is that the deprotonation process of the OEC proceeds before the electron transfer, and the O–O bond formation occurs >250 μs after the third photo-excitation, in agreement with previous studies [7] , [17] , [46] , [47] . Structural changes that are large enough to access with the current XRD resolution of 4.5–5.2 Å were not observed in the OEC, surrounding amino acid residues, or the quinone sides on the S 3 , S 3 Y Z ox ’ and S 0 state formation, which implies that the structural changes in the OEC are within the order of ≤0.5 Å. Interestingly, our RT structural data clearly show the presence of several features—although not interpretable at the present resolution—in the mF o –DF c difference electron density maps, indicating structural differences in the RT XFEL data compared with the previous SR cryogenic structural models. Future improvements in the crystal quality and data, especially the anomalous signal, will also allow us to use the XFEL approach to resolve the sequence of the important structural and electronic changes during the S 3 → S 3 Y Z ox → S 4 → S 0 transition, providing unprecedented experimental insights into the mechanism of photosynthetic water oxidation. Sample preparation PS II was purified from T. elongatus as described elsewhere [48] . Crystals that were obtained as described in ref. 48 and a seed kit (Hampton Research, CA, USA) were used to produce a PS II seed stock solution in buffer A (100 mM PIPES, pH 7, 5 mM CaCl 2 , 6% (w/w) PEG 2000, 0.03% β-dodecyl maltoside) for microcrystallization of PS II. Microcrystals of PS II were obtained by mixing aliquots of the PS II seed stock solution with PS II solution (chlorophyll (Chl) concentration 4 mM, corresponding to a protein concentration of~40 mg ml −1 ) in a 1:4 ratio. Box-shaped crystals (5–10 μm in the longest dimension, 5 μm in the shorter dimension) were suspended in buffer C (100 mM MES, pH 6.5, 5 mM CaCl 2 , 10% (w/v) PEG 2000, 30% (w/v) glycerol). The final concentration of the crystal suspension was determined by measuring Chl concentration of small aliquots of the suspension, dissolved in 80% acetone [49] . The Chl concentration was adjusted between 0.3 and 0.5 mM, corresponding to a protein concentration of 8.5–14 μM (3–5 mg ml −1 ). For solution samples, the purified PS II was resuspended in buffer D (100 mM MES, pH 6.5, 5 mM CaCl 2 , 0.015% β-dodecyl maltoside, 1.3 M sucrose) to a final protein concentration of 80–90 mg ml −1 . Thermolysin was obtained from Hampton Research (CA, USA). Microcrystals of thermolysin were obtained as described previously [28] using PEG2000 as a precipitant. MIMS measurements Sample suspensions of PS II from T. elongatus of 8 mg ml −1 Chl were diluted to 7 mg ml −1 Chl with H 2 18 O (98%) to give a final enrichment of H 2 18 O of ~12% and final salt concentrations of 4.4 mM CaCl 2 , 85 mM MES and 1.1 M sucrose. No electron acceptors were added. The 18 O-enriched samples were loaded into a gas-tight Hamilton syringe and pumped through a silica capillary (inner diameter (ID)=50 μm, outside diameter (OD) 160 μm) into another gas tight Hamilton syringe that collected the sample. Both syringes were placed on separate syringe pumps. Samples were kept in darkness or very dim green light during all steps, except when illuminated inside the capillary with laser light travelling through one to four optical fibres (400 μm core diameter) directly attached to a region of the capillary with the polyimide coating removed. This set-up directly mirrors the in-capillary illumination set up for the CXI experiment (see Fig. 1a and below). The oscillation pattern of PS II crystals was obtained in the same way, but the experimental details were as follows: the PS II crystal suspension was concentrated to 3.2 mM Chl and was then diluted with H 2 18 O (98%) to 2.5 mM Chl to give a final enrichment of 21.5%. The final concentrations of other additions were 5 mM CaCl 2 , 80 mM MES, 1.2 M sucrose and 11% PEG 2000. The capillary that was used to conduct these experiments had an ID of 100 μm and an OD of 360 μm. A Nd:YAG laser (Continuum Inlite II-20, 532 nm, 7 ns pulse width) was used for sample illumination. To obtain a stable output intensity of 7 μJ per fibre (intensities of individual flashes may vary by ±5%), the laser was operated continuously at 20 Hz. The illumination periods were set with the help of a fast shutter (SH05 operated with SC10 Controller; both from Thorlabs), while the flash frequency was controlled via the Q-switch divider (20 or 10 Hz). The oxygen produced was quantified by injecting the illuminated sample into a membrane-inlet cell containing 600 μl water, connected via a Si membrane (Mem 213) and a cooling trap (dry ice/ethanol) to an isotope ratio mass spectrometer (DELTA V, ThermoFinnigan) [50] . The O 2 formed during illumination was detected with excellent S/N ratio as the non-labelled 16 O 16 O, the mixed labelled 16 O 18 O and double-labelled 18 O 18 O species. To obtain a flash pattern, the light-induced yields for O 2 production (detected at m/z =34) obtained with ( x −1) illuminations were subtracted from that with x illuminations ( Fig. 2b ). For the first flash, the background 34 O 2 signal of a non-illuminated sample was subtracted. Each measurement was repeated twice (deviation of the points was within 10%). Determination of the total O 2 produced per PS II complex Determination of the total O 2 produced per PS II complex and flash number requires the absolute calibration of the MIMS signals. This calibration was achieved by the injection of known volumes of air-saturated water into the MIMS cell. This value was used to determine the micromoles of O 2 produced by PS II by the illumination with 3 flashes using 7 μJ per fibre measured in a silica capillary (ID=75 μm, OD 160 μm), with a flow rate of 0.5 μl min −1 and a flash frequency of 4 Hz. To account for diffusion losses of 34 O 2 out of the capillary during the flow of the sample, a loss factor was determined separately by measuring the O 2 content of a PS II sample that was illuminated inside a gas tight syringe by 50 consecutive Xenon lamp flashes (2 Hz frequency, in the presence of acceptors) and either directly injected into the MIMS cell or first flowed through the capillary set-up used for the flash measurements into the collection syringe and then injected into the MIMS cell. After correcting the O 2 amount obtained in the 3F experiment by the loss factor, this number was then divided by the μmole of PS II reaction centre, which resulted in ~0.73 O 2 /RC ( Fig. 2a ). As three consecutive flashes are required to produce one molecule of oxygen in a dark-adapted PS II reaction centre, a maximum of one O 2 /reaction centre can be expected under these conditions. The above number of 73% oxygen yield directly translates into light saturation. For 100% light saturation, we would expect a value of 73% (0.9 3 ), as even under stationary conditions an average ‘miss’ of 10% occurs due to charge equillibria within PS II. Sample injection and illumination at CXI Samples were injected into the CXI instrument chamber [32] using an electrospun liquid microjet [28] . Aliquots of 50–150 μl of sample were placed in a microcentrifuge tube placed inside the pressurized cell with a Pt-electrode and the end of the injector capillary submerged in the sample. Pressures of 17–20 psi against the CXI chamber pressure (10 −4 Torr) and voltages of around 3,000 V were applied depending on the buffer composition and crystal concentration. The injector capillary was a clear silica capillary with an ID of 75 or 100 μm and an OD of 150 or 360 μm, respectively. The flow rate was in the range of 0.25–1.0 μl min −1 (for the 75 μm ID capillary) and 1.2–3.5 μl min −1 (for the 100 μm ID capillary) depending on the sample viscosity and the backing pressure. We measured the flow rate from the mass of sample consumed divided by the run time (data quoted here was obtained this way), and in several cases we also estimated the flow rate from the velocity of crystals flowing in the capillary by using in-capillary visualization of the flow via a microscope-mounted camera. To ensure that the samples were in the dark stable S 1 state before injection, all sample handling and storage was performed in darkness or under dim green light. For visualization of the jet, an infrared laser diode (Coherent Lasiris, 785 nm, 15 mW) was used (see ref. 28 for details). The wavelength was chosen to be outside the absorption spectrum of PS II. Sample illumination for advancement into higher S -states was conducted using the output of a frequency-doubled Nd:YLF laser at 527 nm (Coherent Evolution) with 150 ns pulse duration. The light from the laser was coupled into multi-mode fibre light guides with a core diameter of 400 μm. Three of these light guides (laser 1, 2 and 3 in Fig. 1a ) were directly coupled onto the silica capillary of the sample injector and an additional laser (laser 4 in Fig. 1a ) illuminated the sample in the jet. The output of all three fibres was equalized to 10 μJ per pulse (1.4 times the power necessary for saturation of the oxygen production in our offline O 2 f1ash yield experiments, see above) using wave plates, and the transmission profile and output power of all fibres was measured before the experiment and after each change to the experimental set-up. The centre–centre distance between the fibres was 1.98 mm and typical illumination parameters for a 75-μm ID capillary (1 μl min −1 flow rate, 8.9 Hz illumination frequency) result in a delay between the pump laser flashes on the same volume segment of 0.52 s. To generate 2F samples (enriched in the S 3 state), lasers 2 and 3 were used, and the sample reached the X-ray interaction region ~0.5 s after the second pump laser flash. To generate 3F samples (enriched in the S 0 state), lasers 1, 2 and 3 were used and the sample reached the X-ray interaction region ~0.5 s after the third pump laser flash. Finally, to study transients during the S 3 to S 0 transition, lasers 2 and 3 (for advancing the sample from the S 1 to the S 3 state) in combination with laser 4 (to start the transition from the S 3 to the S 0 state) were used. In this experiment, the time delay of the X-ray probe with respect to the laser 4 was set to 250 μs, giving rise to the 3F′ data (enriched in the S 3 Y Z ox state). CXI instrument and X-ray parameters The CXI instrument of LCLS [32] was used in the 1-μm focus setting with the beam being focused to 1.5 × 1.5 μm 2 full-width half maximum using Kirkpatrick–Baez mirrors [51] . The pulse length used was ~45 fs and the repetition rate was 120 Hz. The energy was varied between 7.1 and 9.7 keV with 3–6 × 10 11 photons per pulse. The dose therefore varied between 50 and 300 MGy. XES was measured using 7.1 keV excitation, due to the higher cross section for the Mn transition at this energy. XRD of PS II was measured at both energies but no difference in diffraction quality between the two energies was observed. The majority of the PS II XRD data was obtained with incident energy of 7.1 keV. XRD of thermolysin was collected at 9.7 keV (above the Zn edge). X-ray emission spectroscopy setup X-ray emission spectra were recorded in a shot-by-shot mode using a custom-built spectrometer in the von Hamos geometry [25] , [52] . The crystal analyser array was located 500 mm from the interaction point and with an angle of 81° between the centre of the array and the X-ray beam. A set of 16 Si(440) crystal analysers was used and the Bragg angle range was 85.9° to 83.4°, equivalent to an energy range from 6,473.8 to 6,500 eV (limited by the detector size). The signal was recorded on a 140 k CSPAD [53] , [54] , located below the interaction region. The set-up was calibrated by recording spectra from solutions of Mn II Cl 2 as previously described [25] . The first moment values of the emission spectra were calculated between 6,486 and 6,494 eV as described [35] . Before computing difference spectra, the flash state spectra were smoothed by using either a moving average over a 0.5-eV window or by fitting a cubic polynomial of 3 eV width to each data point. SR XES spectra were recorded at European Synchrotron Radiation Facility (ESRF) beamline ID 26 using the 440 reflection of five spherically bent ( R =1,000 mm) Si crystal analysers in combination with a silicon drift detector aligned in a Rowland geometry. The overall energy bandwidth of the X-ray emission spectrometer was 0.8 eV. The sample was kept at 15 K in a liquid He cryostat surrounded by He as a heat-exchange gas. The ESRF storage ring was run in 16 bunch mode with ring currents between 60 and 90 mA. The incident beam was monochromatized and tuned to 6.75 keV using the 111 reflection of a pair of cryogenically cooled Si crystals. The beam size was 1.0 (h) × 0.2 (v) mm 2 and the beam position on the sample was changed after 1 s of X-ray illumination. Computational facilities Over a 5-day period, 114-TB data were collected at LCLS, grouped into five 12-h shifts. Data were processed immediately to assess their completeness and quality. However, as the data size exceeded the processing capacity of the 480-core Linux cluster available at LCLS, arrangements were made to access an additional 1,000 Linux cores at the National Energy Research Scientific Computing Center (NERSC). Transfer of the data from SLAC to NERSC was made over the Energy Sciences Network at a maximum sustained rate of 7.5 Gb s −1 . XRD data processing XRD data were recorded using the large CSPAD at LCLS’s CXI instrument [32] , and processed using cctbx.xfel [55] , [56] . A dark-current image (pedestal) was subtracted from each image before data reduction. An initial triage step was evaluated, retaining only those images containing 16 or more strong, low-resolution Bragg spots as determined by the Spotfinder procedure [56] , [57] . However, it was found that this step rejected some useful data; thus, it was ultimately omitted from the data processing protocol. Indexing (determination of the unit cell and crystal orientation) was performed with the LABELIT implementation [58] of the Rossmann DPS algorithm [59] , [60] , and was guided by supplying the known unit cell [61] , [62] . Where more than one crystal was exposed in the same shot, indexing was attempted on the two most dominant lattices [56] . The number of images or lattices retained after each processing step is detailed in Supplementary Table 1 . Crystal orientations determined by LABELIT were optimized by minimizing the positional difference between the observed Bragg spots and those predicted by the model. Orientational models were further refined so that minimal perturbations were needed to exactly fit the observed Bragg spots to Bragg’s law, under the simplifying assumptions of a perfect crystal lattice and a monochromatic beam. Differences between this idealized model and the actual set of observations then allowed us to estimate crystal properties such as mosaicity and the average size of coherently scattering mosaic blocks, leading to a realistic model of Bragg spot positions suitable for signal integration. Intensities were integrated by summation within a spot mask derived from nearby strong spots atop a planar background [63] , [64] and corrected for polarization [65] . Intensity variances, σ 2 ( I ), were derived by counting statistics [66] and a coarse estimate of the detector gain. Error estimates from each diffraction pattern were then inflated by assuming that negative values of I /σ( I ) are actually decoy measurements (noise only) with a Gaussian distribution centred at zero and with an s.d. of 1, thus providing a lower bound on modelling errors. A separate resolution cutoff was determined for each image based on a Wilson plot (average intensity versus binned resolution). Integrated, non-negative intensities from separate images were then scaled to intensities derived from isomorphous reference structures (PDB codes 3bz1 and 3bz2 for PS II [12] and PDB code 2tli for thermolysin [37] ), without separately accounting for the partiality fraction of each observation. Images whose intensities correlated poorly (≤10%) with those of the reference model were rejected, as were images that deviated from the reference unit cell lengths (10%) or angles (2°), or that did not obey the expected symmetry. Multiple measurements with the same Miller index were merged by averaging and the error was modelled by propagating the σ ( I ) values in quadrature. The resolution cutoff for the merged data sets was determined from the resolution dependence both of the multiplicity and of CC 1/2 , the correlation coefficient of semi-data sets merged from odd- and even-numbered images [36] . The expected contribution of the anomalous signal to |F| was estimated using the Web server of the Biomolecular Structure Center at University of Washington ( http://skuld.bmsc.washington.edu/scatter/AS_index.html ). Phasing and refinement As a starting PSII model, we used PDB IDs 3bz1 and 3bz2 (ref. 12 , modified to include all atoms in the OEC based on the high-resolution structure 3arc [13] , and re-refined against the 3bz1/3bz2 deposited amplitudes in phenix.refine [67] . The structure was then reduced to a single copy of the PS II complex and the processed data sets were phased by molecular replacement in Phaser [68] . Refinement of coordinates and B-factors was performed in phenix.refine using tight restraints, including two-fold non-crystallographic symmetry, with the distances between heavy atoms in the OEC restrained to the values determined by EXAFS [20] . Simulated annealing omit maps were generated with the OEC atoms set to zero occupancy, with harmonic restraints [69] applied to the OEC and surrounding atoms; the default parameters of a starting temperature of 5,000K and 100 K steps were used. Isomorphous difference maps were generated using phenix.fobs_minus_fobs_map . Structures and maps were aligned using the PHENIX structure comparison tool. All structure figures were created in PyMOL 1.2. The thermolysin structure was solved by molecular replacement using PDB ID 2tli [37] with metals and waters removed, rebuilt using the PHENIX AutoBuild wizard [70] and refined in phenix.refine . Simulated annealing omit maps were generated as for PS II, with Zn and Ca occupancies set to zero. Accession codes: The X-ray crystallographic coordinates and structure factors for structures reported in this study have been deposited at the Protein Data Bank (PDB), under deposition numbers 4TNL (thermolysin), 4TNH (PS II dark state), 4TNJ (PS II 2F), 4TNI (PS II 3F) and 4TNK (PS II 3F’). These data can be obtained free of charge from www.pdb.org . How to cite this article: Kern, J. et al. Taking snapshots of photosynthetic water oxidation using femtosecond X-ray diffraction and spectroscopy. Nat. Commun. 5:4371 doi: 10.1038/ncomms5371 (2014).